Protruding Pt single-sites on hexagonal ZnIn2S4to accelerate photocatalytic hydrogen evolution Single-site cocatalysts engineered on supports offer a cost-efficient pathway to utilize precious metals, yet improving the performance further with minimal catalyst loading is still highly desirable. Here we have conducted a photochemical reaction to stabilize ultralow Pt co-catalysts (0.26 wt%) onto the basal plane of hexagonal ZnIn 2 S 4 nanosheets (Pt SS -ZIS) to form a Pt-S 3 protrusion tetrahedron coordination structure. Compared with the traditional defect-trapped Pt single-site counterparts, the protruding Pt single-sites on h -ZIS photocatalyst enhance the H 2 evolution yield rate by a factor of 2.2, which could reach 17.5 mmol g −1 h −1 under visible light irradiation. Importantly, through simple drop-casting, a thin Pt SS -ZIS film is prepared, and large amount of observable H 2 bubbles are generated, providing great potential for practical solar-light-driven H 2 production. The protruding single Pt atoms in Pt SS -ZIS could inhibit the recombination of electron-hole pairs and cause a tip effect to optimize the adsorption/desorption behavior of H through effective proton mass transfer, which synergistically promote reaction thermodynamics and kinetics. Water splitting for hydrogen (H 2 ) generation through solar light has attracted increasing attention since it supplies a significant carbon-neutral technology for zero-emission renewable energy evolution. The design of a photocatalyst with high efficiency and long durability is a focused task for researchers to scale up H 2 evolution reaction (HER) in the past decades [1] . Two-dimensional (2D) hexagonal ZnIn 2 S 4 ( h -ZIS), a typical ternary chalcogenide with favorable H adsorption features at edge S atom in (110) facet ( \(\Delta {G}_{{{{{{\rm{H}}}}}}}^{* }\) = −0.16 eV) and robust resistance to photocorrosion, has been regarded as a promising candidate for photocatalytic water splitting [2] , [3] , [4] , [5] , [6] . The current guiding principles for advancing the catalytic performance of h -ZIS are as follows. First, increase the active site density in h -ZIS through preferentially exposing the edge sites [6] , [7] . Unfortunately, unleashing the intrinsically high activity of h -ZIS is still retarded by the severe recombination of electron-hole pairs, where only a small quantity of electrons could survive at the active sites. Second, create in-plane sulfur vacancies or dope metallic heteroatoms to substitute Zn atoms [7] , [8] , [9] , [10] . The lifetime of photoexcited electrons is prolonged, and the basal-plane S atoms in those h -ZIS are also stimulated as centers for HER; however, these S sites suffer from less favorable hydrogen adsorption features ( \(\Delta {G}_{{{{{{\rm{H}}}}}}}^{* }\) = −0.25 eV) despite the increased site density [9] . Apparently, h -ZIS only becomes applicable toward photocatalytic HER when the rapid carrier recombination and limited active site obstacles are simultaneously overcome. As a lamellar material, the basal plane of h -ZIS provides plenty of platforms for noble-metal nanoparticles loading, especially platinum (Pt), while the scarcity and high cost of the noble-metal co-catalysts tremendously inhibit their large-scale implementation [2] , [11] , [12] , [13] . Alternatively, single-site co-catalysts (SSCs) emerge as a frontier for catalysis science due to their high atom efficiency and outstanding activity [14] , [15] . The strong metal-support interaction caused by metal atoms and coordinated atoms would affect the charge distributions and introduce the electronic structure modifications, which influence the electron-hole pairs recombination and the adsorption behavior during the catalytic process, and eventually change their catalytic activity and selectivity [16] , [17] , [18] , [19] . One of the effective strategies for advanced SSCs is to produce more active sites through increasing metal loading with no aggregation, and accordingly, several Pt single-site (Pt SS )-based photocatalysts (Pt loading with 8.7 wt% [20] or 12.0 wt% [21] ) have exhibited exciting H 2 evolution rate and observable bubbles under visible light irradiation. For practical applications, achieving maximum catalytic performance with minimal noble-metal atoms is essentially required. Recently, Pt SSCs supported on highly curved substrates were successfully prepared as electrocatalyst to mimic the metal sites at the edges and corners of particles [22] . Owing to the accumulation of electrons around Pt regions triggered by the tip effect, an accelerated HER kinetics was achieved. Principally, the generation of tip enhancement is biased onto curvature-rich configurations (typically corner, vertex, or protrusion) [23] . To this end, direct anchoring Pt SSCs onto h -ZIS nanosheets might be an effective approach to form tridimensional protrusion that could produce high- and cost-efficient photocatalysts for HER. In this work, a photochemical route was employed to synthesize h -ZIS with Pt single sites (Pt SS -ZIS) [24] . The light-induced reaction is more moderate and controllable than traditional annealing methods, so the structure of h -ZIS could be well preserved without generating any vacancy defects. During photochemical processes, PtCl 6 2− ions were reduced and concurrently immobilized on the basal plane of h -ZIS nanosheets, forming Pt–S 3 tetrahedron coordination structure with surrounding S atoms. Experiments and simulations jointly manifest that the atomically dispersed Pt atoms could serve as sinks to facilitate the separation of photoexcited electron-hole pairs as well as active centers to enhance the HER performance through the accelerating catalytic kinetics. As a result, the synergetic effect of atomic-level Pt and h -ZIS produces a higher photocatalytic activity for H 2 evolution, where the activity outperforms that of defect-trapped Pt single-site counterpart. In addition, a thin film of Pt SS -ZIS on the solid substrate could readily be achieved through a drop-casting approach, and a large amount of H 2 bubbles are generated during light irradiation (Supplementary Movies 1 and 2 ). Structure analysis and characterization Ultrathin h -ZIS nanosheets with thickness ranging from 2.46 to 4.94 nm were prepared by a hydrothermal method (Supplementary Fig. 1 ) [9] . H 2 PtCl 6 aqueous solution was introduced into h -ZIS dispersion with magnetic stirring. The interfacial charges of h -ZIS and Pt species (HPtCl 6 − or PtCl 6 2− ) were opposite, so they would be spontaneously assembled through electrostatic interaction in the solution, with Pt-ZIS mixture generated (Supplementary Fig. 2 ). After irradiation under visible light for 60 min, Pt sites were immobilized on h -ZIS, and the mixture was centrifuged and collected (see the Experimental Section and Supplementary Fig. 3 ). 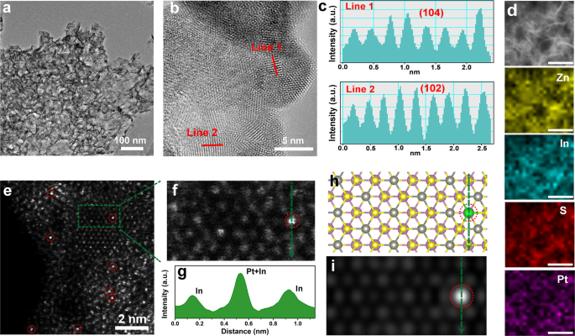Fig. 1: Structural characterization of Pt0.3-ZIS. aTEM image of Pt0.3-ZIS.b,cHRTEM image of Pt0.3-ZIS.dElemental mapping of Pt0.3-ZIS. The scale bars are 50 nm.eHAADF-STEM image of Pt0.3-ZIS.fMagnified HAADF-STEM image of Pt0.3-ZIS.gStrength profiles from the areas labeled by green line.hOptimized structure of Pt0.3-ZIS. The yellow, gray, pink, and green spheres represent the S, Zn, In, and Pt atom, respectively.iSimulated HAADF-STEM image of PtSS-ZIS according to DFT-optimized structure. By alerting the volume of added H 2 PtCl 6 , Pt loading content could be tuned, as quantified by the inductively coupled plasma optical emission spectroscopy (ICP-OES) analysis (Supplementary Table 1 ). Additionally, the molar ratio of Zn and In in Pt 0.3 -ZIS was calculated to be 0.225:0.451, which is consistent with the theoretical molar ratio of 1:2. X-ray diffraction (XRD) patterns and Raman spectra with negligible changes are observed between h -ZIS and Pt-ZIS, suggesting that Pt atoms incorporation does not destroy the crystal structure of h -ZIS (Supplementary Fig. 4 ). Transmission electronmicroscopy (TEM) and high-resolution TEM (HRTEM) images in Supplementary Fig. 5 depict a sheet-like structure of h -ZIS and the lattice fringe of 0.41 nm corresponds to the (006) facet. After Pt deposition, the obtained Pt-ZIS nanosheets maintain the thickness (3.10–5.11 nm) of pristine h -ZIS recorded by atomic force microscope (AFM) (Supplementary Figs. 6 and 7 ). As shown in TEM and HRTEM images, no Pt nanoparticles are observed with Pt loading content in the range of 0.1–1.4 wt%, and the energy-dispersive X-ray spectroscopy (EDS) also exhibits homogeneous dispersion of Pt on h -ZIS nanosheets without any aggregation (Fig. 1a–d and Supplementary Figs. 8 – 10 ). When further increasing the Pt amount to 3.0 wt%, nanoparticles were formed, which is proved by the green circles and corresponding EDS spectrum (Supplementary Fig. 11 ). In addition, the lattice fringe of 0.293 and 0.196 nm attribute to the h -ZIS (104) and Pt (200) facet, respectively. To reveal the configuration of Pt co-catalyst on h -ZIS nanosheets, aberration-corrected high angle annular dark field STEM (HAADF-STEM) measurements were carried out on h -ZIS and Pt 0.3 -ZIS. Since the contrast in HAADF-STEM image is proportional to the square of atomic number, Pt is much brighter than Zn, In, and S atoms, and the atomically dispersed bright spots (circled) in Fig. 1e and Supplementary Fig. 12 confirm the formation of single Pt atoms [25] . On the contrary, no bright spots could be observed in h -ZIS, and the cross-sectional profiles of atom contrast show almost identical intensity (Supplementary Fig. 13 ). As a result, the cross-sectional intensity in Fig. 1f and g , together with the ICP-OES results and electron spin resonance (ESR) spectra (Supplementary Fig. 14 ), directly identify that Pt SSCs exist, not as interior dopants substituting for Zn or In in h -ZIS skeletons, but as external adatoms conjugating with h -ZIS to engender tridimensional protrusions, different from extensively reported planar geometry of metal-N x - and defect-trapped-SSCs [13] , [26] . To illustrate the exact position of Pt single sites, density functional theory (DFT) calculations were carried out to determine the energies of Pt atoms on various sites. Six different locations were established, including Zn-S hollow site, Zn atop, S atop on Zn-S plane, In-S hollow site, In atop, and S atop on In-S plane, respectively, and Zn-S hollow site with the largest adsorption energy is confirmed to be the most stable location for Pt atom occupation (Supplementary Figs. 15 – 17 ). The distribution of Pt atoms on h -ZIS and their propensity to agglomerate was also examined by calculating the energy difference between an isolated Pt atom and a Pt dimer (Δ E d ), in which the total energy of the isolated configuration was used as reference energy. As shown in Supplementary Fig. 18 , it is more favorable for the Pt atoms to be isolated at Zn-S hollow site due to the positive Δ E d of 2.03 eV, which fully supports the experimental observations of the Pt single atom in Pt 0.3 -ZIS. Based on the DFT-optimized structure, a STEM simulation on Pt SSCs dispersed h -ZIS was performed. The simulated result is in good agreement with the experimental HAADF-STEM image, demonstrating that Pt single sites prefer to chemisorb above the Zn-S hollow site in h -ZIS basal plane (Fig. 1h and i ). Fig. 1: Structural characterization of Pt 0.3 -ZIS. a TEM image of Pt 0.3 -ZIS. b , c HRTEM image of Pt 0.3 -ZIS. d Elemental mapping of Pt 0.3 -ZIS. The scale bars are 50 nm. e HAADF-STEM image of Pt 0.3 -ZIS. f Magnified HAADF-STEM image of Pt 0.3 -ZIS. g Strength profiles from the areas labeled by green line. h Optimized structure of Pt 0.3 -ZIS. The yellow, gray, pink, and green spheres represent the S, Zn, In, and Pt atom, respectively. i Simulated HAADF-STEM image of Pt SS -ZIS according to DFT-optimized structure. Full size image Electronic states of atoms in Pt-ZIS Elemental composition and chemical states of Pt-ZIS were characterized by X-ray photoelectron spectroscopy (XPS). The high-resolution Zn 2p and In 3d XPS peaks corresponding to h -ZIS, Pt 0.3 -ZIS, and Pt 3.0 -ZIS exhibit little shift (Supplementary Fig. 19 ). The S 2p spectrum for h -ZIS shows two peaks at 161.8 and 163.0 eV, respectively. After loading Pt single sites, a blue-shift of ~0.4 eV in Pt 0.3 -ZIS is observed, indicating that the electrons are transferred from Pt to h -ZIS and enriched around S atom. This also proves that the decoration of Pt single atoms would modulate the electronic structures of h -ZIS (Fig. 2a ) [20] , [27] . With the increasing amount of Pt to 3.0 wt%, a smaller blue-shift of about 0.3 eV is detected. For the Pt 4 f spectra, Pt/C exhibits three peaks at 71.90, 71.77, and 73.19 eV, which correspond to the Pt 0 , Pt 2+ , and Pt 4+ state, respectively (Fig. 2b ) [16] . In contrast, the Pt 0.3 -ZIS mainly contains Pt δ+ species (72.10 eV), revealing the formation of a higher coordination number with the Pt–S bonds than the Pt–Pt bonds [28] , [29] , [30] . Interestingly, both Pt 0 and Pt δ+ peaks appear in the spectrum of Pt 3.0 -ZIS (70.90 and 72.09 eV), which is probably owing to the well-constructed both Pt single atoms and nanoparticles [29] . The detailed information for XPS fits is listed in Supplementary Tables 2 – 5 . Fig. 2: Electronic states of atoms in photocatalysts. a High-resolution XPS spectra (S 2p ) of h -ZIS, Pt 3.0 -ZIS, and Pt 0.3 -ZIS. b High-resolution XPS spectra (Pt 4 f ) of Pt/C, Pt 3.0 -ZIS, and Pt 0.3 -ZIS. c Fourier transform of k 2 -weighted Pt L 3 -edge of the EXAFS spectra for Pt foil, PtO 2 , Pt 1.4 -ZIS, and Pt 3.0 -ZIS. d Wavelet transform for the k 2 -weighted EXAFS spectra of Pt foil, PtO 2 , Pt 1.4 -ZIS, and Pt 3.0 -ZIS. R is the interatomic distance. FTIR spectra of CO adsorbed after the desorption processes for e h -ZIS, f Pt 0.3 -ZIS, and g Pt 3.0 -ZIS. Full size image Furthermore, X-ray absorption near-edge structure (XANES) and extended X-ray absorption fine structure spectroscopy (EXAFS) were conducted to investigate the local atomic structure and electronic environment of Pt species in Pt-ZIS. EXAFS results in Fig. 2c show k 2 -weighted Fourier transforms from the Pt L 3 -edge EXAFS oscillations of Pt 1.4 -ZIS and Pt 3.0 -ZIS in comparison to that of Pt foil and PtO 2 ( k 2 -weighted χ( k ) signals in Supplementary Fig. 20 ). The only prominent shell in Pt 1.4 -ZIS locating at near 2.0 Å without any Pt–Pt contribution in the range of 2–3 Å testifies the atomically dispersed Pt on h -ZIS [17] , [29] , whereas an additional peak at about 2.6 Å arises in Pt 3.0 -ZIS, closing to that of Pt–Pt contribution. To gain visual illustrations of Pt coordination conditions, wavelet transform (WT) of the k 2 -weighted EXAFS spectra, a reflection of structure information in the resolution of R space and K space, are shown in Fig. 2d . Pt 1.4 -ZIS exhibits the maximum WT intensity at 1.8–2.1 Å in R space and 3–6 Å in k space, ascribing to Pt–S bond in the first coordination shell [31] , [32] . While a new WT intensity maximum near 2.5–2.8 Å and 9–11 Å suggests the coexistence of Pt–S and Pt–Pt bonds in Pt 3.0 -ZIS. The Fourier-transform EXAFS curves and the corresponding fitting results in Supplementary Fig. 21 and Supplementary Table 6 give the Pt–S coordination number of 2.6 for Pt 1.4 -ZIS, implying a similar coordination condition of Pt–S 3 in Pt SS -ZIS as depicted by HAADF-STEM image and DFT simulations. The XANES spectra of Pt L 3 -edge show that the white-line intensity of Pt 1.4 -ZIS is lower than that of PtO 2 , but higher than that of Pt 3.0 -ZIS and Pt foil, demonstrating the Pt atoms are in an oxidation state originating from covalent Pt–S bonds, which is consistent with XPS results (Supplementary Fig. 22 ) [19] . Moreover, we investigated the CO adsorption behavior on different photocatalysts using Fourier-transform infrared (FTIR) spectroscopy to provide additional information about the dispersion and chemical state of Pt (Fig. 2e–g ). For Pt 0.3 -ZIS, only a weak vibration band appears at 2093 cm −1 corresponding to CO adsorption on Pt δ+ [33] , [34] . While the adsorption of CO also produces a strong vibration band at 2033 cm −1 and another weak band at 1961 cm −1 for Pt 3.0 -ZIS. The main band at 2033 cm −1 can be ascribed to linearly bonded CO on Pt 0 sites, and the band at 1961 cm −1 is caused by CO adsorbed on the interface between Pt clusters and the support [33] . All these characterizations provide compelling evidence that our protocol affords Pt 0.3 -ZIS with only positively charged Pt single atoms, while Pt 3.0 -ZIS with both single atoms and Pt nanoparticles. Photocatalytic H 2 evolution performances With protrusion-shaped SSCs in hand, we next explored their photocatalytic HER activities in an aqueous solution with 10 vol% triethanolamine (TEOA) as the sacrificial agent under visible light ( λ > 420 nm) irradiation. According to Fig. 3a , all Pt-loaded h -ZIS photocatalysts exhibit higher H 2 evolution performance than the counterpart ( h -ZIS: 19.67 μmol h −1 with 20 mg photocatalyst). The optimized rate (350.1 μmol h −1 ) is acquired at Pt 0.3 -ZIS, which is about 17.8 times enhanced than that of pristine h -ZIS. When Pt loading content exceeds 0.3 wt%, the activity experiences a decrease, and the catalytic efficiency of each Pt site is reduced (Supplementary Fig. 23 ). In addition, h -ZIS with sulfur vacancies ( h -ZIS-V S ) was synthesized through the treatment of NaBH 4 in a water bath. Benefiting from the existence of localized states caused by sulfur vacancies, h -ZIS-V S performs a narrower bandgap (2.66 eV) and a longer average fluorescence lifetime (5.86 ns) than h -ZIS (2.79 eV and 3.02 ns) (Supplementary Figs. 24 and 25 ). As a result, the photocatalytic activity of h -ZIS is enhanced after creating sulfur vacancies. Then Pt 0.3 -ZIS-V S (0.28 wt% Pt) was also prepared by the same photochemical procedure (Supplementary Fig. 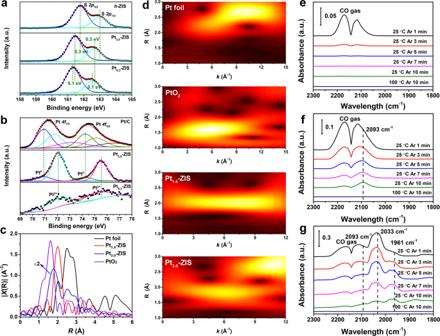Fig. 2: Electronic states of atoms in photocatalysts. aHigh-resolution XPS spectra (S2p) ofh-ZIS, Pt3.0-ZIS, and Pt0.3-ZIS.bHigh-resolution XPS spectra (Pt4f) of Pt/C, Pt3.0-ZIS, and Pt0.3-ZIS.cFourier transform ofk2-weighted Pt L3-edge of the EXAFS spectra for Pt foil, PtO2, Pt1.4-ZIS, and Pt3.0-ZIS.dWavelet transform for thek2-weighted EXAFS spectra of Pt foil, PtO2, Pt1.4-ZIS, and Pt3.0-ZIS.Ris the interatomic distance. FTIR spectra of CO adsorbed after the desorption processes foreh-ZIS,fPt0.3-ZIS, andgPt3.0-ZIS. 26 ). The obviously decreased ESR signal of Pt 0.3 -ZIS-V S and the calculated adsorption energy reveal that Pt single atoms incline to be trapped at defect sites rather than protrude out of h -ZIS-V S surface (Supplementary Figs. 26 , 27 ). The recorded H 2 generation rate for Pt 0.3 -ZIS-V S is only about half of that for Pt 0.3 -ZIS (Fig. 3 b). These results imply that the excellent catalytic activity of Pt 0.3 -ZIS could be mainly attributed to the protrusion-like Pt species on 2D h -ZIS. Similar to the trend of visible light, Pt 0.3 -ZIS also displays a boosted activity under simulated solar light with a total H 2 generation of 3504 μmol within 6 h, whereas only 245.7 μmol H 2 is formed by h -ZIS (Supplementary Fig. 28 ). Additionally, Pt 0.3 -ZIS could introduce acceptable HER performance even in pure water and the H 2 evolution rate is ~24.04 μmol h −1 (1202 μmol h −1 g −1 ) under visible light irradiation (Supplementary Fig. 29 ). Dependence of apparent quantum efficiency (AQE) at each wavelength for Pt 0.3 -ZIS derived from the amount of generated H 2 was estimated by various band-pass filters (Fig. 3c and Supplementary Table 7 ). The AQE matches well with the absorption spectrum of Pt 0.3 -ZIS, and reaches up to 50.4% at 420 nm. Experiments in dark or without photocatalysts show no H 2 evolution, demonstrating that H 2 is generated by the photocatalysis processes. Such high AQE and catalytic HER activity of Pt 0.3 -ZIS is far beyond the majority of representative photocatalysts (details see the comparisons in Fig. 3d and Supplementary Table 8 ). Furthermore, Pt 0.3 -ZIS almost maintains its photocatalytic H 2 evolution rate at the initial level after continuous irradiation for 50 h (Fig. 3e ). The characterizations including XRD, XPS, TEM, and HAADF-STEM, demonstrate that the structures undergo negligible changes, manifesting high stability of Pt 0.3 -ZIS (Supplementary Figs. 30 – 33 ). Fig. 3: Evaluation of photocatalytic HER performances. a Visible light ( λ > 420 nm) photocatalytic H 2 evolution activities of h -ZIS and Pt-ZIS with different Pt loading content. b Visible light ( λ > 420 nm) photocatalytic H 2 evolution activity of Pt 0.3 -ZIS in comparison with h -ZIS, h -ZIS-V S , and Pt 0.3 -ZIS-V S . c Wavelength dependen c e of the AQE for Pt 0.3 -ZIS. d H 2 evolution rates for Pt 0.3 -ZIS in this work compared with representative recently reported photocatalysts. e Cycling stability t e st of Pt 0.3 -ZIS. f , g Digital photograph of H 2 evolution using Pt 0.3 -ZIS film without and with visible light irradiation. Full size image Due to its outstanding performance, we dispersed Pt 0.3 -ZIS into ethanol solution and then drop-casted onto FTO substrate (1.5 × 2 cm 2 ) to form a thin film (~3 μm thick) with excellent transmittance (Supplementary Figs. 34 and 35 ). As a proof-of-concept, the resultant Pt 0.3 -ZIS film was employed as a photocatalyst for H 2 production. No H 2 is generated before irradiation, while small H 2 bubbles start to appear continuously when turning on the light (Fig. 3f, g and Supplementary Movies 1 , 2 ). The H 2 generation rate over the film achieves as high as 0.967 L h −1 m −2 (43.17 mmol h −1 m −2 ) under visible light irradiation, outperforming numerous recent reported photocatalysis films, such as C 3 N 4 film (0.19 L h −1 m −2 ) and Pt SS -MOF (0.398 L h −1 m –2 ), which dictates an enormous potential for real applications [21] , [35] . Insight of the increased photocatalytic activity To shed light on the origin of enhanced activity, three elementary processes in photocatalysis HER, namely light absorption, charge separation, and interfacial H 2 catalysis, are taken into consideration. The optical absorption properties were examined by ultraviolet-visible (UV-vis) diffuse reflectance spectra. An absorption edge at around 440 nm corresponding to the bandgap of about 2.85 eV, is observed for Pt 0.3 -ZIS. It is slightly larger than that of pristine h -ZIS (2.79 eV), revealing a blue-shift absorption edge of h -ZIS upon Pt stabilizing (Fig. 4a and b ). These results are similar to those achieved from the photocurrent action spectra of different photocatalysts film electrodes (Supplementary Fig. 36 ). Even though the light absorption is enhanced in the visible range with further increasing the amount of Pt (Pt 3.0 -ZIS), the measured photocurrent action spectrum of Pt 3.0 -ZIS is quite different from its UV-vis absorbance, in which there is almost no photocurrent at 500 nm. Additionally, the AQE of Pt 3.0 -ZIS was also recorded (Supplementary Fig. 37 and Table S7 ). Consistent with the photocurrent action, the AQE of Pt 3.0 -ZIS does not follow well with the UV-vis spectrum and only a little amount of H 2 is generated at 500 nm. Considering that the Pt colloids exhibit broadband optical absorption from ultraviolet to the visible light region, we can conclude that Pt nanoparticles formed in Pt 3.0 -ZIS could extend the light absorption, but have limited contributions to the photocatalytic performances of h -ZIS [36] . The digital images demonstrate an obvious color change from ivory to pale yellow for h -ZIS and Pt 0.3 -ZIS, and finally to dark brown for Pt 3.0 -ZIS. The relationship between VBM, E f , and E vac , and the UPS spectra of different photocatalysts are shown in Fig. 4c . The vacuum level ( E vac ) should be located 21.2 eV above the cutoff energy ( E cutoff ) of the spectrum. The relative locations of valence band maximum (VBM) are calculated to be −6.14 eV ( h -ZIS) and −6.12 eV (Pt 0.3 -ZIS) compared with E vac according to UPS spectra (Fig. 4d ). As a result, h -ZIS and Pt 0.3 -ZIS display the conduction band minimum (CBM) potential of −3.35 and −3.27 eV, respectively (Fig. 4e ). The detailed band positions are illustrated in Supplementary Table 9 . The elevation of CBM endows the photoexcited electrons in Pt 0.3 -ZIS with a higher reduction ability to react with hydrogen ions and form molecular hydrogen in HER compared with h -ZIS [4] . This favorable feature of the band structure is advantageous to prohibit the recombination of electron-hole pairs, and is responsible for the enhanced photocatalytic performance of Pt 0.3 -ZIS. Fig. 4: Mechanism insight the photocatalytic H 2 evolution. a UV–vis diffuse reflectance spectra for h -ZIS, Pt 0.3 -ZIS, and Pt 3.0 -ZIS, insert: digital images for h -ZIS, Pt 0.3 -ZIS, and Pt 3.0 -ZIS, the concentration of suspensions is 2 mg mL −1 . b Bandgap for h -ZIS and Pt 0.3 -ZIS. c Comparison and relationship of VBM, E f , and E vac of UPS spectra. d UPS spectra of h -ZIS and Pt 0.3 -ZIS in the valence band region. e Schematic illustration of the band structure of h -ZIS and Pt 0.3 -ZIS. f Normalized time profiles of transient absorption at 1150 nm during the TDR of h -ZIS, Pt 0.3 -ZIS, and Pt 3.0 -ZIS. Full size image The electron dynamics involved in photocatalysis were revealed by time-resolved diffuse reflectance (TDR) spectroscopy, a robust technique to provide direct evidence for the effect of Pt loading on charge separation in semiconductors [37] , [38] . The pump light with a central wavelength of 420 nm was used, which is effective for photoinduced an interband transition in h -ZIS. It turns out that probing in the wavelength range of 900–1200 nm yielded similar TDR spectra, featuring free or trapped photoexcited electrons (Supplementary Fig. 38 ) [6] , [39] , [40] . And a set of representative data obtained at 1150 nm combined with the biexponential fitting results are illustrated. In Fig. 4f , the two-time constants for h -ZIS are τ 1 = 12.5 ps (52.7%) and τ 2 = 567 ps (47.3%), respectively, and the weighted average lifetime is 554 ps. In comparison, the characterized two-time constants for Pt 0.3 -ZIS (τ 1 = 0.259 ps (97.0%) and τ 2 = 16.6 ps (3.0%)) and Pt 3.0 -ZIS (τ 1 = 0.782 ps (89.2%) and τ 2 = 31.6 ps (10.8%)) lead to much shorter average lifetime of 11.1 and 26.4 ps, respectively. In general, the average recovery lifetime is considered as a crucial indicator for evaluating the separation efficiency of photoexcited electron-hole pairs, and such a shortened lifetime indicates the opening of an additional pathway for electron transfer after Pt deposition [41] , [42] . Based on the mean transient decay times of h -ZIS ( τ ZIS ), Pt 0.3 -ZIS ( τ 0.3 ), and Pt 3.0 -ZIS ( τ 3.0 ), we can determine the injection rate through the equation as \({k}_{{{{{{\rm{ET}}}}}}}=(1/{{\tau }}_{x})-(1/{{\tau }}_{{{{{{\rm{ZIS}}}}}}})\) , where x represents the weight ratio of Pt [43] , [44] . It is calculated that the k ET of Pt 0.3 -ZIS is 8.8 × 10 7 s −1 , to be ~2.4 times faster than that of Pt 3.0 -ZIS (3.6 × 10 7 s −1 ). In addition, as a more significant parameter for photocatalytic activity, the efficiency of electron injection ( η inj ) from h -ZIS to Pt is calculated as \({{\eta }}_{{{{{{\rm{inj}}}}}}}=1-{{\tau }}_{x}/{{\tau }}_{{{{{{\rm{ZIS}}}}}}}\) [43] , [44] , and Pt 0.3 -ZIS affords a higher η inj ( η inj = 98.0%) than that of Pt 3.0 -ZIS ( η inj = 95.2%). Additionally, steady-state photoluminescence (PL) spectra were recorded (Supplementary Fig. 39 ). Loading Pt onto h -ZIS results in significant PL quenching for Pt-ZIS, and Pt 0.3 -ZIS exhibits the lowest PL intensity among the photocatalysts, demonstrating an improvement in charge separation [45] . Concurrently, the photocurrent intensity of Pt 0.3 -ZIS is around 6.5 and 3.9 times compared with that of h -ZIS and Pt 3.0 -ZIS, respectively (Supplementary Fig. 40a ). EIS Nyquist plots of h -ZIS, Pt 0.3 -ZIS, and Pt 3.0 -ZIS together with simulated equivalent electrical circuits are also provided in Supplementary Fig. 40b and c , respectively, in which R ct is interfacial charge-transfer resistance [46] . Based on the model, Pt 0.3 -ZIS shows the smallest semicircle diameter and R ct value (Supplementary Table 10 ), proving the lowest resistance of interfacial charge transfer in Pt 0.3 -ZIS [47] . The efficient charge separation in Pt 0.3 -ZIS was also confirmed by photocatalytic activation of peroxymonosulfate (PMS) to degrade antibiotic ornidazole (ONZ) pollutants (Supplementary Fig. 41 ). For Pt 0.3 -ZIS, the degradation efficiency of ONZ is 1.8 and 1.7 times and the utilization efficiency of PMS is 2.4 and 1.8 times than h -ZIS and Pt 3.0 -ZIS, respectively. The effective electrons injection from Pt 0.3 -ZIS to PMS molecules generate more reactive species, contributing to the higher photocatalytic performance than h -ZIS and Pt 3.0 -ZIS. These results disclose that more rapid and efficient directional migration of photogenerated electrons is realized by isolated Pt atoms decoration, partly accounting for Pt 0.3 -ZIS with the greatly enhanced photocatalytic performance [38] , [48] . DFT calculations were further carried out to dive fundamental insight into the effect of atomical Pt decoration. The charge density difference isosurface images reveal a strong charge redistribution at Pt-bonding region after the presence of protrusion-like single Pt atom on the basal plane of h -ZIS, and the calculated Bader charge shows that 0.06 e is transferred from Pt to S atoms in the h -ZIS substrate, confirming the strong interaction between Pt and h -ZIS (Fig. 5a and b ) [30] . It is also observed that the Pt–S 3 coordination has obvious charge transfer along the z direction. When the Pt adsorbate hybridizes with the p band of S, the adsorbate state split into localized bonding and antibonding states. In the projected density of states (PDOS) profile for Pt SS -ZIS, the dominant feature is Pt 5d -S 3p bonding resonances below the Fermi level and forming hybridized electronic states (Fig. 5c ). Such states are considered as the electron acceptor states that could endow Pt SS -ZIS with metallic conductive character to inhibit the recombination of electron-hole pairs [49] . Moreover, the antibonding states of Pt SS -ZIS with the position all above the Fermi level involve in constructing conduction band, which probably leads to the upshift of CBM [19] . This enlarged bandgap for Pt SS -ZIS is consistent with the UV-vis absorption spectra and UPS spectra. Hence, theoretical calculations suggest that the covalent Pt–S coordination bond within Pt SS -ZIS forms additional charge-transfer channels to improve the charge mobility, causing an enhanced photocatalytic activity. Fig. 5: Density functional theory (DFT) calculations. a Top and b side view of calculated charge difference surfaces of Pt SS -ZIS with yellow and cyan colors represent positive and negative electron density isosurfaces, respectively. The value of isosurface is 0.002e/bohr [3] . c Density of states of the h -ZIS and Pt SS -ZIS. d Calculated adsorption energies of H atoms as a function of the H coverages (from one H atom to four H atoms) on the single Pt atom photocatalysts with h -ZIS as support. The H–H and Pt–H distances are shown in the figure. The adsorption energies (E a ) were calculated by: \({{{{{{\rm{E}}}}}}}_{{{{{{\rm{a}}}}}}}=\left[{{{{{{\rm{E}}}}}}}_{{{{{{{\rm{Pt}}}}}}}_{{{{{{\rm{SS}}}}}}}-{{{{{\rm{ZIS}}}}}}}+\frac{{{{{{\rm{n}}}}}}}{2}{{{{{{\rm{E}}}}}}}_{{{{{{{\rm{H}}}}}}}_{2}}-{{{{{{\rm{E}}}}}}}_{{{{{{{\rm{Pt}}}}}}}_{{{{{{\rm{SS}}}}}}}-{{{{{\rm{ZIS}}}}}}+{{{{{\rm{nH}}}}}}}\right]/{{{{{\rm{n}}}}}}\) . The yellow, gray, pink, green, and purple spher e s represent the S, Zn, In, Pt, and H atoms, respectively. e Side view of Pt SS -ZIS schematic structure with one H atom, two H atoms, three H atoms, and four H atoms chemisorbed on Pt atom, termed as H 1,ads Pt-ZIS, H 2,ads Pt-ZIS, H 3,ads Pt-ZIS, and H 4,ads Pt-ZIS, respectively. Full size image To disclose the underlying interfacial catalytic contribution of H 2 O to H 2 from Pt single site, the adsorption of H atom on Pt atom was investigated. It is demonstrated that the adsorption strength of H decreases with an increase in the number of adsorbed H atoms, eventually leading to a minimum value when four H atoms are adsorbed (Fig. 5d ). The single H atom exhibits adsorption energy ( E a ) of 0.613 eV, while it decreases to 0.564 eV per H in the case of two H atoms. As the number of interacting H atoms increases, the Pt to H interaction for bond formation becomes a compromise between the H–H electrostatic repulsion and the orbital hybridization of Pt–H [50] . Specifically, when three H atoms adsorb onto a single Pt atom, they locate symmetrically around Pt site, leading to corresponding adsorption energy of 0.543 eV per H. With the number of H atoms reaching four, the adsorption configuration is one in which a H 2 dimer and two isolated H atoms are formed with an adsorption energy of 0.436 eV per H (Fig. 5d and e ). The bond length of Pt–3H is elongated from 1.551 to 1.746 Å, and that of Pt–4H is 1.723 Å, which are much longer than that of Pt-1H (1.567 Å) and Pt-2H (1.566 Å) (the detailed distance of H–H atoms and Pt–H atoms are labeled in Fig. 5d ). Moreover, the distance between 3H and 4H is only 0.881 Å, close to that in H 2 molecule (0.740 Å). These phenomena indicate the weakened adsorption strength of 3H and 4H on Pt single site, thus promoting the desorption of 3H and 4H and ease of H 2 production on Pt atom. Finally, we performed the H adsorption free energy ( \(\Delta {G}_{{{{{{\rm{H}}}}}}}^{* }\) ) to examine the HER activity for different sites and the number of H atoms. Our simulations indicate that the adsorbed H on Pt, neighboring S, neighboring Zn, and second-neighboring Zn move to the tilted top site toward adjacent Zn atom on the surface after relaxation with an identical \(\Delta {G}_{{{{{{\rm{H}}}}}}}^{* }\) of −0.36 eV, and the \(\Delta {G}_{{{{{{\rm{H}}}}}}}^{* }\) of second-neighboring S is 0.61 eV (Supplementary Figs. 42 , 43 , and Table 11 ). Furthermore, the \(\Delta {G}_{{{{{{\rm{H}}}}}}}^{* }\) gradually increases for the second (−0.26 eV) and third (−0.23 eV) adsorbed H atoms on Pt single site, and it becomes positive for the fourth adsorbed H atom (+0.10 eV) (Supplementary Fig. 44 ). Commonly, one material is regarded as a good HER catalyst when the value of \(\Delta {G}_{{{{{{\rm{H}}}}}}}^{* }\) is close to thermoneutral ( \(\Delta {G}_{{{{{{\rm{H}}}}}}}^{* }\) ≈ 0) [51] . Therefore, we suggest that the Pt single atom would be the active site for HER and the catalyst that forms in situ states might be H 3,ads Pt-ZIS [31] . DFT simulations were also carried out on Pt SS -ZIS-V S . Unlike Pt SS -ZIS, H atom tends to be adsorbed right above Pt atom after structural relaxation, suggesting that it is difficult for Pt atom in Pt SS -ZIS-V S to adsorb more H atom (Supplementary Fig. 45 ). Additionally, the calculated \(\Delta {G}_{{{{{{\rm{H}}}}}}}^{* }\) for H atom on Pt SS -ZIS-V S is -0.22 eV, which is larger than that of H 3,ads Pt SS -ZIS (+0.10 eV). These results prove the recently reported tip enhancement effect that protrusion-like single atoms could continuously enrich protons, which issues an improvement in proton mass transfer, thus boosting the kinetics of H 2 production on the Pt single atom [22] , [26] , [50] , [52] . Active blocking experiment by introducing thiocyanate ion (SCN −1 ) into the catalyst system dictates a drastically decreased H 2 generation rate from 350.1 to 27.44 μmol h −1 with the increase of KSCN concentration, confirming that Pt single atoms indeed serve as the centers for HER (Supplementary Fig. 46 ). Based on calculations, the adsorbed Pt single sites onto the surface of h -ZIS manifests a fast formation and release of molecular hydrogen, leading to an outstanding catalytic activity. By combining experimental results with theoretical calculations, the high catalytic performance of Pt 0.3 -ZIS accompanied with long durability is confirmed. The enhanced H 2 generation rate is due to the atomic protrusion-like Pt atoms with triple roles in the photocatalytic HER. First, single Pt atoms immobilized onto h -ZIS could tune the band structure of h -ZIS on upshifting the CBM, providing a larger reduction driving force. Second, the atomically dispersed Pt are acted as electron wells to accelerate charge separation and transportation. Third, the tridimensional protrusions induce effective proton mass transfer to the active Pt site and an almost thermoneutral \(\Delta {G}_{{{{{{\rm{H}}}}}}}^{* }\) for HER, which is also supported by the smallest overpotential of Pt 0.3 -ZIS among J–V curves (Supplementary Fig. 47 ). A reasonable photocatalytic mechanism for HER from water is proposed (Supplementary Fig. 48 ). Upon light irradiation, the electron and hole pairs are generated and then migrate from the interior to the surface of h -ZIS. Due to the covalent Pt–S coordination bond, electrons are injected from the neighboring S atoms into Pt single atoms efficiently, followed by the reaction with adsorbed protons to generate H 2 . Simultaneously, the holes in h -ZIS are consumed by TEOA. In summary, compared to the conventional defect-trapped-SSCs, atomically dispersed Pt sites are immobilized onto the basal plane of h -ZIS nanosheets to generate catalysts by a facile photochemical strategy. The efficient water reduction activity over Pt 0.3 -ZIS proceeds via regulated band structure, improved charge separation, reduced H 2 evolution overpotential, and advanced protons mass transfer. The demonstration herein of constructing tridimensional protrusions through immobilizing ultralow content Pt SSCs onto 2D h -ZIS nanosheets presents a promising, cost- and energy-efficient avenue for boosting photocatalysis H 2 evolution, and this prototype potentially would stimulate innovative ideas of enabling future ambient HER catalysts of industrial interest. The phenomenon of triggering tip enhancement by high-curvature nano-textures could function as a general prescription to enhance the performances of catalysts achieved in other reactions, such as organic pollutants degradation, O 2 reduction, CO 2 reduction, and N 2 fixation. Synthesis of hexagonal ZnIn 2 S 4 ( h -ZIS) nanosheets In a typical synthesis, 68 mg ZnCl 2 (Aladdin, 99.95%), 293 mg InCl 3 ·4H 2 O (Aladdin, 99.9%), and 300 mg trisodium citrate (Aladdin, 99.0%) are dissolved into 25 mL of deionized water and 5 mL of glycol (Shanghai LingFeng Chemical Reagent Co. LTD., AR). After being drastically stirred for 30 min at room temperature, 150 mg thioacetamide (TAA, SCR, AR) is then added into the solution. After another 30 min stirring, the heterogeneous solution was transferred into a 50 mL Teflon-lined stainless steel autoclave and maintained at 120 °C for 12 h in an oven. After natural cooling, the products were collected by centrifugation, rinsed two times with ethanol and distilled water, and then freeze-dried. Synthesis of hexagonal ZnIn 2 S 4 thin layers with S-vacancy ( h -ZIS-V S ) The as-obtained h -ZIS (100 mg) was dissolved into 50 mL storage bottle containing 0.1 M NaBH 4 (Sinopharm Chemical ReagentCo., Ltd, AR). The mixture was heated at 60 °C in a water bath. After 5 min, the resultant dispersion was centrifuged, and then freeze-dried. Synthesis of Pt-loaded h -ZIS and h -ZIS-V S atomic layers (Pt-ZIS and Pt-ZIS-V S ) In a typical procedure of photochemical loading Pt on h -ZIS, 20 mg thin layers h -ZIS and different amounts of H 2 PtCl 6 (4 mg mL −1 ) were dispersed in an aqueous solution containing 45 mL H 2 O and 5 mL triethanolamine (TEOA, XiLong Scientific, AR). Subsequently, the suspension is bubbled with argon gas through the reactor for 30 min to completely remove the dissolved oxygen and ensure that the reactor is in an anaerobic condition. 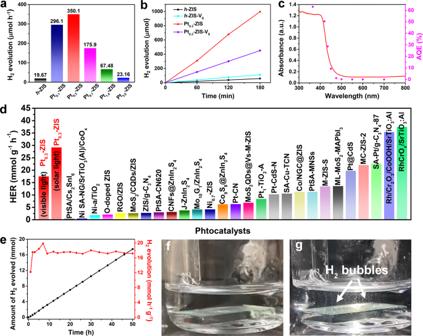Fig. 3: Evaluation of photocatalytic HER performances. aVisible light (λ> 420 nm) photocatalytic H2evolution activities ofh-ZIS and Pt-ZIS with different Pt loading content.bVisible light (λ> 420 nm) photocatalytic H2evolution activity of Pt0.3-ZIS in comparison withh-ZIS,h-ZIS-VS, and Pt0.3-ZIS-VS.cWavelength dependence of the AQE for Pt0.3-ZIS.dH2evolution rates for Pt0.3-ZIS in this work compared with representative recently reported photocatalysts.eCycling stability test of Pt0.3-ZIS.f,gDigital photograph of H2evolution using Pt0.3-ZIS film without and with visible light irradiation. The dispersion was kept stirring with a magnetic stirrer during visible light irradiation ( λ > 420 nm). After the light treatment for 60 min, the sample was centrifuged and washed by deionized water twice and then freeze-dried. By alerting the volume of H 2 PtCl 6 solution, the Pt content relative to h -ZIS was adjusted to about 0.1, 0.3, 0.7, 1.4, and 3.0 wt%, which were named as Pt 0.1 -ZIS, Pt 0.3 -ZIS, Pt 0.7 -ZIS, Pt 1.4 -ZIS, and Pt 3.0 -ZIS, respectively. For the synthesis of Pt 0.3 -ZIS-V S , the procedure was similar to that of Pt 0.3 -ZIS except changing h -ZIS to h -ZIS-V S . 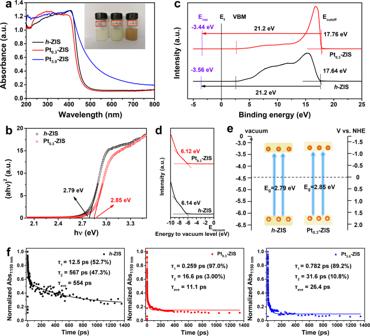Fig. 4: Mechanism insight the photocatalytic H2evolution. aUV–vis diffuse reflectance spectra forh-ZIS, Pt0.3-ZIS, and Pt3.0-ZIS, insert: digital images forh-ZIS, Pt0.3-ZIS, and Pt3.0-ZIS, the concentration of suspensions is 2 mg mL−1.bBandgap forh-ZIS and Pt0.3-ZIS.cComparison and relationship of VBM,Ef, andEvacof UPS spectra.dUPS spectra ofh-ZIS and Pt0.3-ZIS in the valence band region.eSchematic illustration of the band structure ofh-ZIS and Pt0.3-ZIS.fNormalized time profiles of transient absorption at 1150 nm during the TDR ofh-ZIS, Pt0.3-ZIS, and Pt3.0-ZIS. 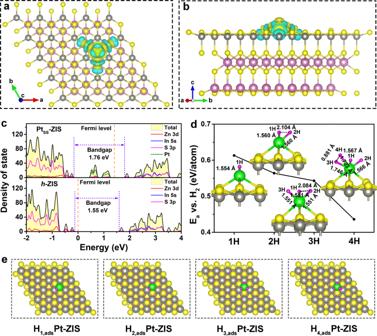Fig. 5: Density functional theory (DFT) calculations. aTop andbside view of calculated charge difference surfaces of PtSS-ZIS with yellow and cyan colors represent positive and negative electron density isosurfaces, respectively. The value of isosurface is 0.002e/bohr3.cDensity of states of theh-ZIS and PtSS-ZIS.dCalculated adsorption energies of H atoms as a function of the H coverages (from one H atom to four H atoms) on the single Pt atom photocatalysts withh-ZIS as support. The H–H and Pt–H distances are shown in the figure. The adsorption energies (Ea) were calculated by:\({{{{{{\rm{E}}}}}}}_{{{{{{\rm{a}}}}}}}=\left[{{{{{{\rm{E}}}}}}}_{{{{{{{\rm{Pt}}}}}}}_{{{{{{\rm{SS}}}}}}}-{{{{{\rm{ZIS}}}}}}}+\frac{{{{{{\rm{n}}}}}}}{2}{{{{{{\rm{E}}}}}}}_{{{{{{{\rm{H}}}}}}}_{2}}-{{{{{{\rm{E}}}}}}}_{{{{{{{\rm{Pt}}}}}}}_{{{{{{\rm{SS}}}}}}}-{{{{{\rm{ZIS}}}}}}+{{{{{\rm{nH}}}}}}}\right]/{{{{{\rm{n}}}}}}\). The yellow, gray, pink, green, and purple spheres represent the S, Zn, In, Pt, and H atoms, respectively.eSide view of PtSS-ZIS schematic structure with one H atom, two H atoms, three H atoms, and four H atoms chemisorbed on Pt atom, termed as H1,adsPt-ZIS, H2,adsPt-ZIS, H3,adsPt-ZIS, and H4,adsPt-ZIS, respectively. Preparation of Pt 0.3 -ZIS thin films Typically, Pt 0.3 -ZIS (30 mg) powder was dispersed into ethanol (2 mL) and then sonicated for 10 min to obtain a colloidal solution. The film was prepared by drop-casting 400 μL of the colloidal solution onto roughened glass (1.5 × 2 cm 2 ). Then the film was dried in a vacuum oven at the temperature of 60 °C. Photocatalytic hydrogen production Twenty milligrams of photocatalysts was dispersed in 45 mL aqueous solution containing 10 vol% TEOA using an ultrasonic bath. Subsequently, the suspension was bubbled with argon gas through the reactor for 30 min to completely remove the dissolved oxygen and ensure that the reactor was in an anaerobic condition. The samples were irradiated under visible light using a 300 W Xenon lamp for H 2 generation (PLS-SXE300D, Beijing Perfectlight Technology Co., Ltd, 300 mW cm −2 ). The reaction temperature is kept at about 8 °C. The visible light is filtered with a nominal 420 nm cutoff filter. The volume of H 2 was measured by Shimadzu GC-8A gas chromatograph equipped with an MS-5A column and thermal conductivity detector. The apparent quantum efficiency (AQE) was calculated using the following equation, 
    AQE ( %)=N_e/N_p×100 % =2×n_H_2×N_A×h×c/S×P×t×λ×100 %
 (1) where N p is the total incident photons, N e is the total reactive electrons, \({n}_{{H}_{2}}\) is the amount of H 2 molecules, N A is Avogadro constant, h is the Planck constant, c is the speed of light, S is the irradiation area, P is the intensity of irradiation light, t is the photoreaction time, and λ is the wavelength of the monochromatic light. For the stability test, the photocatalyst was continuously irradiated for 50 h. The turnover frequency (TOF) was calculated according to the following equation: 
    TOF=n_(H_2)/n_(Pt)·τ
 (2)